Stable metal-organic frameworks containing single-molecule traps for enzyme encapsulation Enzymatic catalytic processes possess great potential in chemical manufacturing, including pharmaceuticals, fuel production and food processing. However, the engineering of enzymes is severely hampered due to their low operational stability and difficulty of reuse. Here, we develop a series of stable metal-organic frameworks with rationally designed ultra-large mesoporous cages as single-molecule traps (SMTs) for enzyme encapsulation. With a high concentration of mesoporous cages as SMTs, PCN-333(Al) encapsulates three enzymes with record-high loadings and recyclability. Immobilized enzymes that most likely undergo single-enzyme encapsulation (SEE) show smaller K m than free enzymes while maintaining comparable catalytic efficiency. Under harsh conditions, the enzyme in SEE exhibits better performance than free enzyme, showing the effectiveness of SEE in preventing enzyme aggregation or denaturation. With extraordinarily large pore size and excellent chemical stability, PCN-333 may be of interest not only for enzyme encapsulation, but also for entrapment of other nanoscaled functional moieties. Metal-organic frameworks (MOFs) with large pores or channels are considered to be promising candidates for the immobilization of many catalysts, such as metal complexes, nanoparticles and enzymes [1] , [2] , [3] , [4] . Immobilization is particularly valuable for enzymes, since they are costly and can be difficult to reuse and recover [5] . A range of solid supports have been explored for enzymes, such as sol gels, hydrogels, organic microparticles, and porous or non-porous inorganic supports [5] . However, there have been disadvantages associated with these supports, including very low protein loading in the non-porous systems and denaturation of enzymes in sol gels due to their brittle and disordered structures [5] , [6] , [7] , [8] , [9] . Mesoporous silica nanoparticles, which have a large pore size, high porosity and a very ordered structure, have been demonstrated as promising enzyme supports [5] . However, due to their one-dimensional (1D) channel structure, insufficient interactions between the inner channel surface of mesoporous silica and enzymes result in significant leaching during multiple cycles of use. Moreover, aggregation still occurs inside the channel [5] , [6] , [7] , [8] , [9] . Recently, we studied MOFs containing predesigned single-molecule traps (SMTs) for carbon capture, wherein each SMT can trap one CO 2 molecule [10] . If the same concept is applied in enzyme immobilization, we can potentially diminish leaching and encapsulate each enzyme molecule in a SMT to eliminate aggregation, optimizing the catalytic environment. MOFs, which have ultra-high porosity, tunable pore shape and size and adjustable surface functionality, are an ideal platform for this novel single-enzyme encapsulation (SEE) or multiple-enzyme encapsulation (MEE) approach. On the basis of structural rationalization, we herein report facile syntheses of a series of highly stable SMT-containing MOFs based on trivalent metal species, namely PCN-332(M) (M=Al(III), Fe(III), Sc(III), V(III), In(III)) and PCN-333(M) (M=Al(III), Fe(III), Sc(III)). PCN-333 exhibits the largest cage (5.5 nm) and one of the highest void volumes (3.84 cm 3 g −1 ) among all reported MOFs. PCN-333(Al, Fe) shows high stability in aqueous solutions with pH values ranging from 3 to 9, making it an extraordinary candidate for enzyme encapsulation. Three enzymes with different sizes, horseradish peroxidase (HRP), cytochrome c (Cyt c ) and microperoxidase-11 (MP-11), were selected. From a pure size-match point of view, HRP and Cyt c will most likely undergo SEE, whereas MP-11 will go through MEE due to size mismatch. Nevertheless, all three enzymes have been successfully encapsulated into PCN-333(Al) with extremely high loading amounts among all reported solid supports. These immobilized enzymes either maintain or surpass their catalytic activities over the free enzymes, and exhibit smaller K m and better catalytic performance in organic solvents. These immobilized enzymes show almost no leaching during catalysis and recycling, and maintain high catalytic activity. Custom-designed synthesis of PCN-332 and PCN-333 The largest pore reported in MOFs was based on a 1D hexagonal channel structure, which requires a complicated synthetic process to make an extremely long organic linker to reach enzymatic size [3] . Considering the structural feature of the 1D channel, it can only partially interact with immobilized enzymes even if the size is very compatible. As is in mesoporous silica, once the enzymes are incorporated, aggregation still exists. Moreover, after those channels are occupied, there is no other pathway allowing the fast diffusion of both reactants and products. In comparison, cages will act as SMTs affording strong interactions between the cages and the encapsulated enzymes. In addition, cages usually have small windows, which can efficiently encapsulate enzymes, diminishing aggregation, eliminating leaching and optimizing the catalytic environment. Unfortunately, there are very few reported MOFs with enzyme compatible cages, and even fewer can survive in aqueous media [3] , [11] , [12] . Thus, MOFs with larger cages and better stability are highly desired for enzyme encapsulation. The extension of organic linkers, which mostly serve as the faces or edges of pores in MOFs, is the main approach to achieve large pores in MOFs [3] , [13] , [14] , [15] , [16] , [17] , [18] , [19] . However, the pore shape or symmetry plays a very important role in determining the overall pore size. Approximating the cross-section of a pore (cage or channel) as a regular polygon with n edges ( Fig. 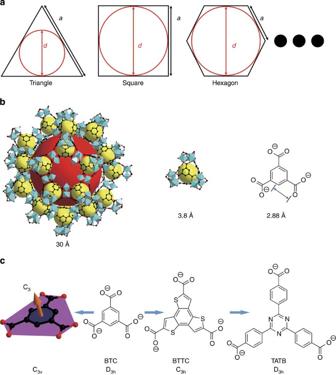Figure 1: Pore expansion with preserved structure (the isoreticular approach). (a) The relationship between the edge (a) and diameter (d) in regular polygons. (b) The largest cage, super tetrahedral unit and organic linker in MIL-100. (c) Idealized symmetries of benzenetricarboxylate (BTC) in MIL-100 and free BTC, BTTC and TATB. 1a ), the diameter d of the inscribed circle corresponding to the pore can be expressed as the following, Figure 1: Pore expansion with preserved structure (the isoreticular approach). ( a ) The relationship between the edge ( a ) and diameter ( d ) in regular polygons. ( b ) The largest cage, super tetrahedral unit and organic linker in MIL-100. ( c ) Idealized symmetries of benzenetricarboxylate (BTC) in MIL-100 and free BTC, BTTC and TATB. Full size image where a is the edge of the regular polygon. If a is considered as the edge of a pore cross-section, then 1/tan ( π / n ) would be the magnification factor, which increases with n and determines how a certain change of a affects the overall pore diameter d . Therefore, by applying the isoreticular approach through ligand extension in MOFs, the pores with larger n values can be more efficiently enlarged than the pores with a smaller n value. Hence, to construct MOFs with ultra-large cages and excellent chemical stability, we applied the isoreticular approach to the chemically highly stable mesoporous MOF, MIL-100 (ref. 20 ). The circular cross-section of the largest cage in MIL-100 is surrounded by 12 supertetrahedra, therefore n is very large ( n =12). In addition, MIL-100 is based on hard Lewis acidic trivalent metal species (Al 3+ , Fe 3+ , Cr 3+ , V 3+ , Sc 3+ ), which interact strongly with carboxylates and give rise to the high stability of the framework in aqueous environments [21] , [22] , [23] , [24] , [25] . Benzenetricarboxylate ( Fig. 1b ), the organic linker in MIL-100, has idealized D 3h symmetry as a free anion. In the framework, the ligand symmetry is reduced to C 3v by a bowl-shaped bending that increases the inherent energy of the ligand (the distance between the two planes is 0.288 Å; Fig. 1c , left). If the symmetry of the free linker were not D 3h , to form a similar structure, the energy of the linker would have been even higher in the framework, making the overall structure extremely energetically unfavored. To guarantee the formation of isoreticular structures of MIL-100, we selected two ligands that are most stable in a trigonal planar conformation, BTTC (benzo-tris-thiophene carboxylate) with a C 3h (pseudo- D 3h in crystallography) symmetry through the fused five-member ring and TATB (4,4’,4’’-s-triazine-2,4,6-triyl-tribenzoate), with idealized D 3h symmetry arised from ligand planarity, which is enforced by conjugation ( Fig. 1c ). Solvothermal reactions of H 3 BTTC or H 3 TATB with MCl 3 (M=Al, Fe, V, Sc, In) afforded octahedral crystals of PCN-332(M) (M=Al, Fe, Sc, V, In) or PCN-333(M) (M=Al, Fe, Sc), respectively ( Fig. 2a , Supplementary Figs 1–16 , Supplementary Data 1 ). High-resolution synchrotron powder X-ray diffraction (PXRD) collected at 17-BM, Argonne National Laboratory shows that PCN-333 is cubic with a≈ 127 Å. This was further confirmed by three-dimensional rotation electron diffraction ( Supplementary Methods and Supplementary Figs 17–20 ). The space group of PCN-333(Al) was determined to be Fd -3 m by combining rotation electron diffraction and high-resolution transmission electron microscopy (HRTEM; Fig. 2c , Supplementary Methods , Supplementary Figs 20,21 ). Structural models of PCN-333 and PCN-332 were built based on the isoreticular structure of MIL-100. The structural models of PCN-333(Al) and PCN-332(Fe) were further refined against the synchrotron PXRD data by Rietveld refinement with soft restraints for the M–O bond distances and rigid body for the ligands ( Fig. 2b and Supplementary Tables 1,2 , Supplementary Fig. 5 ). A two-dimensional map is calculated by an inverse Fourier transformation from the amplitudes and phases of five symmetry-independent reflections with d >14 Å extracted from the HRTEM image ( Fig. 2c,e ), in which channels along the [111] direction with a size around 3.7 nm can be clearly visualized. Owing to the beam damage of the sample and the damping effect of the objective lens (contrast transfer function), amplitudes obtained from the HRTEM image are attenuated. Replacing the amplitudes from the HRTEM image by those from the PXRD pattern gives an improved two-dimensional map ( Fig. 2f ), which matches better the projected potential map of PCN-333(Al) calculated from the structural model ( Fig. 2g ). This strongly indicates that the structural model is correct. 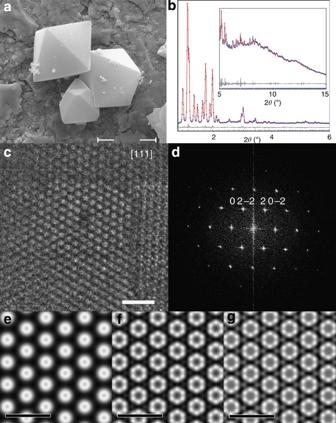Figure 2: Transmission- and scanning electron microscopy anlyses of PCN-333(Al). (a) SEM image of PCN-333(Al). Scale bar, 10 μm; (b) observed (blue), calculated (red) and difference (black) plot for the Rietveld refinement of PCN-333(Al); (c) HRTEM image of PCN-333(Al) taken along the [111] direction, showing the pore with the size of about 3.7 nm in projection. Scale bar, 20 nm; (d) Fourier transform of HRTEM image inc, from which the amplitudes and phases were extracted; (e) Symmetry-averaged map after imposing thep6mmsymmetry on the amplitudes and phases; (f) Symmetry-averaged map (p6mm) calculated using the amplitudes from PXRD and phases from the HRTEM image; (g) Projected electrostatic potential map calculated using the structure factor amplitudes and the phases from the structural model. Scale bars ine–g, 10 nm. Figure 2: Transmission- and scanning electron microscopy anlyses of PCN-333(Al). ( a ) SEM image of PCN-333(Al). Scale bar, 10 μm; ( b ) observed (blue), calculated (red) and difference (black) plot for the Rietveld refinement of PCN-333(Al); ( c ) HRTEM image of PCN-333(Al) taken along the [111] direction, showing the pore with the size of about 3.7 nm in projection. Scale bar, 20 nm; ( d ) Fourier transform of HRTEM image in c , from which the amplitudes and phases were extracted; ( e ) Symmetry-averaged map after imposing the p 6 mm symmetry on the amplitudes and phases; ( f ) Symmetry-averaged map ( p 6 mm ) calculated using the amplitudes from PXRD and phases from the HRTEM image; ( g ) Projected electrostatic potential map calculated using the structure factor amplitudes and the phases from the structural model. Scale bars in e – g , 10 nm. Full size image The structure of PCN-333 is built by sharing the vertices of the supertetrahedra, which consist of M 3 (μ 3 -O)(OH)(H 2 O) 2 units linked along the faces by the organic linkers ( Fig. 3a ). Consequently, two types of mesoporous cages, which can act as SMTs for encapsulation of an enzyme, are generated. A smaller dodecahedral cage is built of 20 supertetrahedra that are connected via vertex sharing to construct a cavity with an exclusive pentagonal window of 25.9 Å in diameter ( Fig. 3b ). A larger hexacaidecahedral (hexagonal-truncated trapezohedral) cage is surrounded by 24 supertetrahedra that form a sphere with not only the pentagonal windows, but also hexagonal windows with a diameter of 30 Å ( Fig. 3b ). The inner diameter is 11 Å for the super tetrahedral cage, 34 Å for the dodecahedral cage and 55 Å for the hexacaidecahedral cage ( Fig. 3b ). The largest cages in PCN-333 lie in a honeycomb arrangement in the [111] projection, which is consistent with the HRTEM result ( Fig. 2 ). PCN-332 exhibits a similar structure as PCN-333, but with smaller cages due to the smaller linker ( Fig. 3 , Supplementary Methods ). 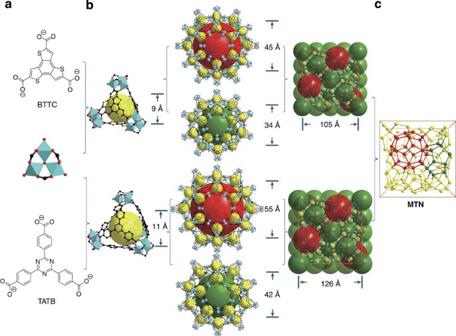Figure 3: Structure illustrations of PCN-332 and PCN-333. (a) Ligands used in PCN-332 and PCN-333. (b) Three different cages in PCN-332 and PCN-333. (c) Simplification of PCN-332 and PCN-333 intoMTNtopology. Figure 3: Structure illustrations of PCN-332 and PCN-333. ( a ) Ligands used in PCN-332 and PCN-333. ( b ) Three different cages in PCN-332 and PCN-333. ( c ) Simplification of PCN-332 and PCN-333 into MTN topology. Full size image Porosity and stability characterization Owing to the small ligand size and strong coordination bond between the organic linker and metal struts, both the PCN-332 and the PCN-333 series can be activated directly on the removal of solvent, while many other MOFs with such high porosity must be carefully activated with supercritical CO 2 (refs 10 , 15 , 16 , 17 , 18 ). To assess the porosity of PCN-332 and PCN-333, we performed Ar sorption at 87 K and N 2 sorption at 77 K ( Fig. 4a,b and Supplementary Figs 22–31 and Supplementary Methods ). PCN-333(Al) shows a total Ar sorption of 2,950 cm 3 g −1 and N 2 uptake of 2,490 cm 3 g −1 . The Brunauer–Emmett–Teller surface area is 4,000 m 2 g −1 . Two steep increases at p / p 0 =0.3 and 0.5 on the Ar adsorption isotherm correspond to two types of mesoporous cages in PCN-333(Al). The experimental void volume of PCN-333(Al) is 3.81 cm 3 g −1 , which is in good agreement with that calculated from the structural model (3.85 cm 3 g −1 ). Such high porosity is comparable to those of the most porous MOFs [13] , [16] , [17] , [18] , [19] , [26] , [27] . The porosity of PCN-333(Fe) is similar to that of PCN-333(Al), while the porosity of PCN-333(Sc) is slightly lower due to its poorer crystallinity. With an isoreticular structure but a smaller organic linker, the porosity and Brunauer–Emmett–Teller surface area of PCN-332 are significantly lower than those of PCN-333. 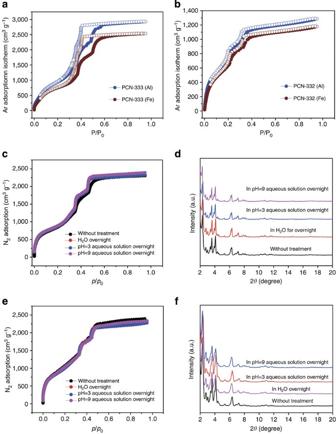Figure 4: Porosity and stability characterization of PCN-333 and PCN-332. (a) Ar sorption isotherms of PCN-333(Fe) and PCN-333(Al); (b) Ar sorption isotherms of PCN-332(Fe) and PCN-332(Al); (c,d) Stability tests of PCN-333(Al); (e,f) Stability tests of PCN-333(Fe). Figure 4: Porosity and stability characterization of PCN-333 and PCN-332. ( a ) Ar sorption isotherms of PCN-333(Fe) and PCN-333(Al); ( b ) Ar sorption isotherms of PCN-332(Fe) and PCN-332(Al); ( c , d ) Stability tests of PCN-333(Al); ( e , f ) Stability tests of PCN-333(Fe). Full size image Despite its high porosity, PCN-333 still shows excellent stability in aqueous solutions. PXRD shows that PCN-333(Al) and PCN-333(Fe) remain intact without loss of crystallinity after immersion in pure H 2 O and in aqueous solutions with pH of 3 and 9 ( Fig. 4d,f ). Furthermore, the N 2 sorption isotherms are almost completely maintained through those treatments ( Fig. 4c,e ), which further demonstrates the stability of these frameworks. The high positive charge density ( Z / r ) on small M 3+ (Al 3+ , Fe 3+ ) ions causes a strong electrostatic interaction between metal nodes and carboxylate linkers, which endows the frameworks with not only excellent stability towards attack by reactive species, but also high thermal stability ( Supplementary Figs 32–39 ). PCN-333(Al) as support for different enzymes PCN-333 is an extraordinary example that meets most prerequisites as a promising enzyme support: the ultra-large cavities can act as SMTs for enzyme encapsulation; the ultra-high porosity ensures high enzyme content after loading which guarantees the overall catalytic efficiency; and the SMTs can efficiently encapsulate enzymes, which can prevent both enzyme aggregation and leaching. In addition, it possesses excellent stability and is compatible with the working environment of an enzyme. A wide variety of enzymes, if smaller than the largest cage (5.5 nm) in PCN-333, can in principle be immobilized [5] . If the enzyme is smaller than the cage, but the cage cannot accommodate two enzymes due to size limitation, a SEE can be achieved. We have selected three commercially available enzymes that are smaller than the largest cage in PCN-333(Al)—HRP, Cyt c and MP-11—for the encapsulation experiment and their catalytic performance and recyclability were also investigated. To the best of our knowledge, all three enzymes have reached record-high loading among all enzyme immobilization cases [5] . The maximum loading is 1.0 g g −1 (22.7 μmol g −1 ) for HRP, 0.95 g g −1 (77.0 μmol g −1 ) for Cyt c and 0.89 g g −1 (478 μmol g −1 ) for MP-11 ( Fig. 5a,b and Table 1 ). Taking into account the size of each enzyme, HRP (size: 4.0 × 4.4 × 6.8 nm) can only be loaded into the large cage, while Cyt c (size: 2.6 × 3.2 × 3.3) is suitable for both the large cage and the medium cage and the small cage with an inner diameter of 1.1 nm will be empty, allowing diffusion of solvent molecules, reactants and products. Assuming SEE, the maximum theoretical loading is 1.27 g g −1 for HRP (assuming only the large cage acts as a SMT) and 1.04 g g −1 for Cyt c (assuming both the large and medium cages act as SMTs), which are in good agreement with the experimental maximum loadings ( Supplementary Methods ). For MP-11, considering its much smaller size (1.1 × 1.7 × 3.3 nm), multiple enzymes may enter each meso-cage, leading to a much higher molar concentration than the other two enzymes. 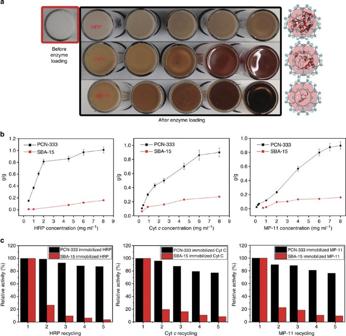Figure 5: Enzyme loading and catalytic recycles of different enzymes. (a) Colour variations of PCN-333(Al) when loaded with different enzymes at different concentrations. (b) Plots of the loading capacities of different enzymes in PCN-333(Al). The standard deviation (error bars) was obtained from three independent replicate experiment. (c) Catalytic activity of immobilized enzymes in each recycle test. Figure 5: Enzyme loading and catalytic recycles of different enzymes. ( a ) Colour variations of PCN-333(Al) when loaded with different enzymes at different concentrations. ( b ) Plots of the loading capacities of different enzymes in PCN-333(Al). The standard deviation (error bars) was obtained from three independent replicate experiment. ( c ) Catalytic activity of immobilized enzymes in each recycle test. Full size image Table 1 Comparison of different enzyme loadings in PCN-333(Al) and SBA-15. Full size table Due to the favourable interaction between the cage and the enzyme, to reach a saturated loading of each enzyme in PCN-333(Al) is rapid. HRP takes about 40 min, Cyt c takes 30 min, while MP-11 takes about 10 min. However, for mesoporous silica, saturated enzyme loading usually takes at least several days to reach [28] , [29] , [30] . After the loading of enzymes, the crystallinity, porosity and thermal stability of PCN-333(Al) samples were characterized, showing well-maintained framework ( Supplementary Figs 40–54 ). Most importantly, the transmission electron microscopy–energy-dispersive X-ray spectroscopy elemental mapping of HRP@PCN-333(Al) sample indicates very well distributed HRP inside of the framework ( Supplementary Fig. 67 ). Enzyme leaching and loss of reactivity on reuse are the major problems for all other enzyme supports [5] . After the immobilization of the three enzymes in PCN-333(Al), their catalytic activity was then evaluated with corresponding reactions ( Supplementary Figs 55–74 ). Oxidation of o-Phenylenediamine catalysed by HRP and oxidation of 2-2’-azino-bis(3-ethylbenzthiazoline-6-sulfonic acid) catalysed by Cyt c and MP-11 were performed, respectively, in acid-sodium citrate buffer with pH=6 at room temperature. Compared with the free enzymes, enzymes immobilized in PCN-333(Al) show relatively smaller k cat values, which may be caused by diffusion control. However, all three enzymes exhibit smaller K m values, resulting in comparable k cat / K m values to the free enzymes ( Table 2 ). The low K m means that the enzyme requires a lower substrate concentration to achieve V max and usually suggests that the enzyme may have a higher affinity with the substrate. Table 2 Comparison of kinetic parameters for free and immobilized enzymes under buffered conditions. Full size table The free enzyme reacts more quickly than the encapsulated enzymes, though it requires significantly more concentration of substrate to reach its peak rate, under carefully controlled conditions designed to prevent it from being aggregated or denatured. However, in practical application, the reaction usually needs to be conducted in different media other than the buffer solution. Therefore, we measured the specific activity to investigate the catalytic activity of SEE and MEE in different media. Cyt c , which is of a suitable size to be incorporated into the two kinds of mesocages in a 1:1 ratio, has most likely undergone SEE, and shows 14 times higher specific activity after immobilization in PCN-333(Al) than the free enzyme in water. To provide a more comprehensive comparison about the immobilized and free Cyt c , the kinetic parameters were investigated in this condition and the results indicate the immobilized Cyt c has a smaller K m , and a higher K cat and K cat / K m in water media ( Table 3 ). Considering that Cyt c suffers severe self-aggregation or denaturation towards temperature or pH variation [31] , such significant catalytic activity enhancement is evidence of SEE in PCN-333(Al). Immobilized HRP, which can also realize SEE, shows slightly higher specific activity ( Supplementary Fig. 68 ) in water. In comparison, MP-11, the size of which is much smaller than the mesocages, suitable for MEE, shows much decreased activity after immobilization ( Supplementary Fig. 68 ). Moreover, in several different organic solvent mixtures, the immobilized HRP performs better than the free HRP ( Supplementary Fig. 71 ). These results show the effectiveness of SEE under harsh reaction conditions. Table 3 Comparison of kinetic parameters for free and immobilized Cyt c in aqueous media. Full size table After the completion of each catalytic reaction, the immobilized enzymes were then recycled by a simple centrifuge. The catalytic reactivity remains almost unchanged for each PCN-333(Al) encapsulated enzyme after several cycles, while very significant decrease of the activity is observed for the same enzymes immobilized in SBA-15, a well-known type of mesoporous silica ( Fig. 5c ). The main reason for the excellent recyclability of PCN-333(Al) immobilized enzymes is the SEE or MEE of these enzymes: there is almost no leaching from these encapsulated enzymes during many cycles while high apparent leaching is observed in SBA-15. Leaching rate is usually thermodynamically related to the interaction strength between the enzyme and the support [5] . Physisorption is usually much weaker than covalent immobilization. However, when there are many interaction sites such as in the case of encapsulation, the overall interaction strength can be stronger than a single covalent bond. Each large cage in PCN-333 is surrounded by many supertetrahedra containing not only highly concentrated metal sites with polarized coordinating water molecules, but also conjugated organic linkers, which generate an amphiphilic inner sphere inside the cage. The cage can therefore act as a SMT, providing a strong trapping interaction to both the hydrophilic and hydrophobic parts of the enzyme, which explains the fast enzyme uptake and the negligible enzyme leaching after encapsulation. The strong interaction between the enzyme and the cages in PCN-333 indicates a large equilibrium constant if the loading process is considered as a reaction. The loading process is less reversible, which leads to fast completion of the forward reaction (enzyme loading). In addition, the small window on each large cage can dynamically reduce the enzyme leaching. In comparison, SBA-15, which has 1D channels with fully hydrophilic surfaces, can provide only limited interaction to immobilized enzymes and lead to very significant enzyme leaching during catalysis and recycling processes. After the encapsulation of enzymes in PCN-333(Al), enzymatic catalysis in organic solvents, an important field in the biotechnological applications of proteins [32] , can be conducted more easily by overcoming the solubility issues for both enzymes in organic media and substrates in aqueous media. The encapsulated HRP shows higher catalytic activity in tetrahydrofuran–water media than it does in pure water, and much higher activity than free HRP under the same condition ( Supplementary Methods ). In summary, by using an exceptionally water-stable MOF containing mesocages that can act as single-molecule traps for the encapsulation of a single-enzyme molecule in one cage, essentially eliminating enzyme aggregation and leaching, immobilized enzymes with recyclability and high catalytic efficiency in harsh condition have been discovered. The single-enzyme encapsulation concept will revolutionize the application of enzymes in industry, enabling the application of enzymes in fundamental processes such as nitrogen fixation, hydrogen production and the conversion of natural gas into liquid fuels of high energy density with unprecedented efficiency. Synthesis of PCN-332(Al) H 3 BTTC (50 mg) and AlCl 3 6H 2 O (200 mg) were dissolved in 10 ml diethylformamide (DEF) or dimethylformamide (DMF), then 1.5 ml trifluoroacetic acid was added. The mixture was heated up at 150 °C in an oven for 12 h until white precipitate formed. The white precipitate was centrifuged and washed with fresh DMF for several times. Yield (based on ligand): ~70%. Synthesis of PCN-332(Fe) H 3 BTTC (50 mg) and anhydrous FeCl 3 (60 mg) were dissolved in 10 ml DEF or DMF, then 1.2 ml trifluoroacetic acid was added. The mixture was heated up at 150 °C in an oven for 12 h until brown precipitate formed. The brown precipitate was centrifuged and washed with fresh DMF for several times. Yield (based on ligand): ~85%. Synthesis of PCN-332(V) H 3 BTTC (50 mg) and anhydrous VCl 3 (60 mg) were dissolved in 10 ml DEF or DMF. The mixture was heated up at 150 °C in an oven for 4 h until green precipitate formed. The green precipitate was centrifuged and washed with fresh DMF for several times. Yield (based on ligand): ~75%. Synthesis of PCN-332(Sc) H 3 BTTC (50 mg) and ScCl 3 6H 2 O (200 mg) were dissolved in 10 ml DEF or DMF. The mixture was heated up at 150 °C in an oven for 4 h until white precipitate formed. The white precipitate was centrifuged and washed with fresh DMF for several times. Yield (based on ligand): ~80%. Synthesis of PCN-332(In) H 3 BTTC (10 mg) and In(NO 3 ) 3 xH 2 O (20 mg) were dissolved in 2 ml DMF, then 0.2 ml HNO 3 (3 M in DMF) was added. The mixture was heated up at 150 °C in an oven for 12 h. The white precipitate was centrifuged and washed with fresh DMF for several times. Yield (based on ligand): ~85%. Synthesis of PCN-333(Al) H 3 TATB (50 mg) and AlCl 3 6H 2 O (200 mg) were dissolved in 10 ml DEF or DMF, then 1.0 ml trifluoroacetic acid was added. The mixture was heated up at 135 °C in an oven for 2 days until white precipitate formed. The white precipitate was centrifuged and washed with fresh DMF for several times. Yield (based on ligand): 80%. Synthesis of PCN-333(Fe) H 3 TATB (50 mg) and anhydrous FeCl 3 (60 mg) were dissolved in 10 ml DEF or DMF, then 0.5 ml trifluoroacetic acid was added. The mixture was heated up at 150 °C in an oven for 12 h until brown precipitate formed. The brown precipitate was centrifuged and washed with fresh DMF for several times. Yield (based on ligand): 85%. Synthesis of PCN-333(Sc) H 3 TATB (50 mg) and ScCl 3 6H 2 O (200 mg) were dissolved in 10 ml DEF or DMF. The mixture was heated up at 150 °C in an oven for 4 h until white precipitate formed. The white precipitate was centrifuged and washed with fresh DMF for several times. Yield (based on ligand): ~85%. How to cite this article : Feng, D. et al . Stable metal-organic frameworks containing single-molecule traps for enzyme encapsulation. Nat. Commun. 6:5979 doi: 10.1038/ncomms6979 (2015). Accession codes: The X-ray crystallographic coordinates for structures reported in this Article have been deposited at the Cambridge Crystallographic Data Centre (CCDC), under deposition number 999752 (PCN-332(Fe)) and 997911 (PCN-333(Al)). These data can be obtained free of charge from The Cambridge Crystallographic Data Centre via www.ccdc.cam.ac.uk/data_request/cif .